Quantum mechanical limit to plasmonic enhancement as observed by surface-enhanced Raman scattering Plasmonic nanostructures enable light to be concentrated into nanoscale ‘hotspots’, wherein the intensity of light can be enhanced by orders of magnitude. This plasmonic enhancement significantly boosts the efficiency of nanoscale light–matter interactions, enabling unique linear and nonlinear optical applications. Large enhancements are often observed within narrow gaps or at sharp tips, as predicted by the classical electromagnetic theory. Only recently has it become appreciated that quantum mechanical effects could emerge as the feature size approaches atomic length-scale. Here we experimentally demonstrate, through observations of surface-enhanced Raman scattering, that the emergence of electron tunnelling at optical frequencies limits the maximum achievable plasmonic enhancement. Such quantum mechanical effects are revealed for metallic nanostructures with gap-widths in the single-digit angstrom range by correlating each structure with its optical properties. This work furthers our understanding of quantum mechanical effects in plasmonic systems and could enable future applications of quantum plasmonics. The interaction between electromagnetic radiation and metallic nanostructures can excite collective oscillations of electrons that are termed localized surface plasmon resonances. These can be supported on many different types of nanostructures, but one design that has proven particularly effective has been that of the plasmonic dimer—two nanoparticles separated by a nanoscale gap [1] . Illumination of a plasmonic dimer with the electric field polarized across the gap results in so called plasmonic ‘hotspots’, wherein light intensity can be enhanced by orders of magnitude over the incident intensity. Such plasmonic enhancements significantly boost the efficiencies of nanoscale light-matter interactions and have enabled applications that include single-molecule detection [2] , [3] , optical manipulation [4] , [5] and nanoscale nonlinear optics [6] , [7] . The mechanism of the plasmonic enhancements has been well studied within the framework of classical electromagnetic theory, which predicts that electric field enhancement increases monotonically as the gap narrows [8] . Only recently has it become appreciated that quantum mechanical effects such as nonlocality [9] , [10] , [11] and electron tunnelling [12] , [13] emerge as the gap-width approaches atomic length-scale. Recent experimental efforts have primarily focused on the impact of these quantum mechanical effects on the far-field radiation properties of plasmonic nanostructures [10] , [14] , [15] , [16] , [17] . Meanwhile, it has been theoretically predicted that they also significantly alter the near-field properties, that is, the field enhancement. Zuloaga et al. [12] , for example, predicted that electron tunnelling reduces the build-up of charges of opposite sign on the two sides of the gap, thereby reducing the maximum achievable field enhancement. However, experimental verification of the quantum mechanical impact on field enhancement, the magnitude of which is directly related to hotspot intensity, has been hindered by difficulties in realizing such small gaps. While there has recently been considerable progress in the fabrication of metallic dimers with angstrom-scale gaps, in some cases there have been difficulties in achieving the tunnelling regime [18] , [19] , while in others the experiments have been unsuitable for measuring field enhancement [15] , [16] , [17] . One optical phenomenon that is strongly related to field enhancement is surface-enhanced Raman scattering (SERS). In SERS, the electromagnetic enhancement of Raman scattering from molecules scales roughly as the fourth power of the local electric field enhancement [20] . SERS enhancement factors, therefore, are likely to be very strongly affected by quantum mechanical modification to plasmonic field enhancement. Here, using small Raman molecules as a probe, we study the impact of quantum mechanical effects on the plasmonic enhancement by observations of SERS. We develop a top-down nanofabrication method that achieves lithographically fabricated plasmonic dimers with gap-widths as narrow as (2.0±0.6) Å, as revealed by high-resolution transmission electron microscopy (TEM). Through correlation between the structural characterization of each individual dimer and its optical properties, we demonstrate that the maximum achievable plasmonic enhancement is limited by quantum mechanical electron tunnelling at optical frequencies. This work is likely to redirect the design considerations of plasmonic nanostructures for linear and nonlinear nanoscale optical applications. It also furthers our understanding of quantum mechanical effects in plasmonic systems and could enable future applications of quantum plasmonics. Fabrication of dimers with angstrom-scale gap-width Top-down fabrication of plasmonic nanostructures traditionally makes use of electron-beam lithography (EBL), evaporation and the lift-off process. This allows flexible design and high yield [21] , but the achievable feature sizes are limited by the resolution of the electron-beam resist and other factors [19] , [22] , [23] . Here, we circumvent this limitation by a two-step EBL process to achieve metallic dimers separated by angstrom-scale gaps ( Fig. 1a , also see Methods). The nanoparticles constituting the dimers are gold discs with diameters of 90 nm and thicknesses of 20 nm, on top of a titanium adhesion layer (1 nm thick). In the first step, the left side of each dimer, along with two alignment marks, is patterned by EBL, followed by evaporation and lift-off. In the second EBL step, the right side of each dimer is patterned, aligned to the left sides using an alignment procedure that corrects offset position (error<10 nm) and rotational angle (error<1 mrad). To account for alignment error, the designed pattern starts from dimers with overlapping features (overlapped by 40 nm) on the lower left corner, to dimers with large gap-widths (40 nm) on the upper right corner. One should therefore expect that while angstrom-scale gaps will not necessarily be achieved at its centre, they will occur at other locations within the array. 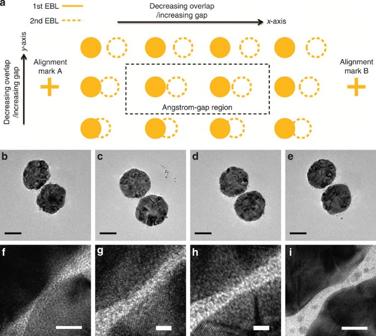Figure 1: Lithographic nanofabrication of dimers with atomic length-scale gap-width. (a) Schematic depiction of the two-step EBL process for the fabrication. Solid objects represent the patterns in the first step. Dashed objects represent the patterns in the second EBL, aligned with the first EBL using a procedure that corrects offset position (error<10 nm) and rotational angle (error<1 mrad). This two-step EBL process generates patterns from dimers with overlapping features (overlapped by 40 nm) on the lower left corner, to dimers with large gap-widths (40 nm) on the upper right corner. Although angstrom-scale gaps will not necessarily be achieved at its centre due to alignment error, they will occur at other locations within the array. (b–e) Top-view: TEM images of four representative Dimers I, II, III and IV with gradually increasing gap-width. The scale bars are 50 nm. (f–i) High-resolution magnified-view TEM images of gap regions of dimers of panels (b–e). In Dimer I, nanoparticles touch; while Dimers II-IV have gap-widths of 2.0 Å, 6.7 Å and 5.8 nm, respectively. The scale bars in (f–i) are 5, 2, 2 and 10 nm, respectively. Figure 1: Lithographic nanofabrication of dimers with atomic length-scale gap-width. ( a ) Schematic depiction of the two-step EBL process for the fabrication. Solid objects represent the patterns in the first step. Dashed objects represent the patterns in the second EBL, aligned with the first EBL using a procedure that corrects offset position (error<10 nm) and rotational angle (error<1 mrad). This two-step EBL process generates patterns from dimers with overlapping features (overlapped by 40 nm) on the lower left corner, to dimers with large gap-widths (40 nm) on the upper right corner. Although angstrom-scale gaps will not necessarily be achieved at its centre due to alignment error, they will occur at other locations within the array. ( b – e ) Top-view: TEM images of four representative Dimers I, II, III and IV with gradually increasing gap-width. The scale bars are 50 nm. ( f – i ) High-resolution magnified-view TEM images of gap regions of dimers of panels ( b – e ). In Dimer I, nanoparticles touch; while Dimers II-IV have gap-widths of 2.0 Å, 6.7 Å and 5.8 nm, respectively. The scale bars in ( f – i ) are 5, 2, 2 and 10 nm, respectively. Full size image To facilitate the characterization of angstrom-scale gaps inside TEM, fabrication is performed on silicon nitride membranes with thicknesses of 30 nm. Figure 1b–e shows top-view TEM images of four fabricated dimers, which are termed Dimers I, II, III and IV, respectively. The gap-widths of the dimers are measured from magnified views of the gap regions shown in Fig. 1f–i . The atomic lattice of gold can be observed from these TEM images, indicating that the resolution is high enough to enable the characterization of the angstrom-scale gaps. Small particles observed around the dimers are produced during metal evaporations and are consistently observed by TEM for similar structures [22] . We select dimers that have no such particles in the smallest region of the gap. To prevent possible parallax [18] arising from sample tilting that could occur due to the high aspect ratio (gold thickness/gap-width) of the dimers, TEM images are taken at 10 additional angles in which the TEM sample holder is rotated within ±30° about an axis in the plane of the substrate and perpendicular to the long axis of the dimers ( Supplementary Fig. 1 ). We analyse each such TEM image and define the gap-width as the distance between the two closest points on the two discs ( Supplementary Fig. 2 and Supplementary Note 1 ). Using this method, the two nanodiscs of Dimer I are found to be touching; the gap-widths for Dimers II and III are estimated to be (2.0±0.6) and (6.7±1.1) Å, respectively, which are comparable to the atomic lattice constant of gold [18] , and the gap-width for Dimer IV is estimated to be 5.8 nm. More examples of dimers with angstrom-scale gap-width are shown in Supplementary Fig. 3 . Identifying electron tunnelling at optical frequencies To demonstrate that the fabricated dimers exhibit quantum mechanical effects, we measure their dark-field scattering spectra (see Methods) and first compare them with the results of classical electromagnetic model (CEM) simulations (see Methods). All optical measurements reported in this paper are performed before TEM characterization to avoid the possibility of carbon contamination. 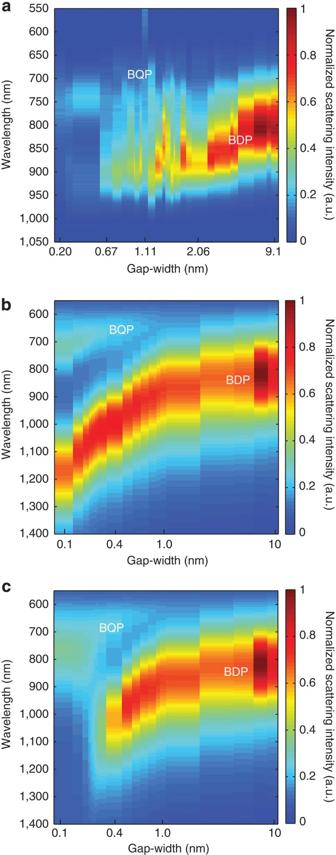Figure 2: Impact of electron tunnelling on dark-field scattering from dimers with angstrom-scale gaps. (a) Measured dark-field scattering spectra from dimers with various gap-widths. Horizontal axis represents measured gap-widths from 9.1 nm to 2.0 Å in log scale. The scattering intensities are normalized by their largest value. (b) Scattering intensities simulated by CEM for gap-widths from 1 Å to 10 nm. The scattering intensities are normalized by their largest value. (c) Scattering intensities simulated by QCM for same range of gap-widths as in panel (b). Again, the scattering intensities are normalized by their largest value. For gap-widths <4 Å, features due to electron tunnelling are observed. These are similar to those of the measured results (panela) for dimers with gap-widths <6.7 Å. Figure 2a shows scattering spectra measured from dimers with gap-widths ranging from 9.1 nm to 2.0 Å. The classical plasmon hybridization theory [24] reveals two resonance modes for the dimers in the wavelength range of interest, namely the bonding dipolar plasmon (BDP) mode and bonding quadrupolar plasmon (BQP) mode, whose charge density distributions are shown in Supplementary Fig. 4 . For gap-widths decreasing from 9.1 nm to 6.7 Å, the measured BDP peak resonance red-shifts from 807 to 892 nm, while the scattering intensity drops to 46% of its peak value. The scattering intensities of the BQP are much weaker than those of the BDP. Meanwhile, CEM simulations predict that, as the gap-width decreases from 10 nm to 7 Å, the BDP peak resonance shifts from 800 to 929 nm, and the scattering intensity drops to 83% of its peak value ( Fig. 2b ). As we discuss below, the drop in the measured scattering intensity is more significant than that predicted by the CEM simulations and can be attributed to the onset of quantum mechanical effects. Nonetheless, the measured peak wavelength of the BDP mode red-shifts monotonically with decreasing gap-width, as predicted by the CEM simulation, suggesting that classical plasmon hybridization is dominant for gap-widths within this range. Figure 2: Impact of electron tunnelling on dark-field scattering from dimers with angstrom-scale gaps. ( a ) Measured dark-field scattering spectra from dimers with various gap-widths. Horizontal axis represents measured gap-widths from 9.1 nm to 2.0 Å in log scale. The scattering intensities are normalized by their largest value. ( b ) Scattering intensities simulated by CEM for gap-widths from 1 Å to 10 nm. The scattering intensities are normalized by their largest value. ( c ) Scattering intensities simulated by QCM for same range of gap-widths as in panel ( b ). Again, the scattering intensities are normalized by their largest value. For gap-widths <4 Å, features due to electron tunnelling are observed. These are similar to those of the measured results (panel a ) for dimers with gap-widths <6.7 Å. Full size image As the gap narrows from 6.7 Å (Dimer III) down to 2.0 Å (Dimer II), very interesting spectroscopic behaviours are observed for the BDP mode around 900 nm in the measured scattering spectra: the scattering resonance peak no longer red-shifts, and the scattering intensity becomes comparable to or even smaller than that of the BQP around 750 nm. These two features in Fig. 2a differ substantially from the prediction of CEM simulations in Fig. 2b . In fact, these two features indicate the emergence of a new charge-transfer plasmon mode that is due to a new ‘charge-transfer' channel in between the two nanodiscs [25] . We first exclude the possibility that such ‘charge-transfer' channel is originated from the adhesion layer. Although the adhesion layers of the two nanodiscs appear to be touching, the simulation results indicate that their conductance is still not large enough to introduce the charge-transfer plasmon mode ( Supplementary Fig. 5 ). To understand the observations in Fig. 2a , we consider a quantum mechanical effect, namely the direct electron tunnelling at optical frequencies across the gap [12] . As the gap-width approaches atomic length-scale, the electron wavefunction on opposite sides of the gap are able to overlap, providing the ‘charge transfer' channel through electron tunnelling. We simulate this effect by adopting the newly developed quantum-corrected model (QCM; see Methods), which allows simulation of electron tunnelling by numerical tools within the classical framework. As shown in Fig. 2c , for gap-widths >4 Å, scattering spectra simulated from QCM simulations reproduce those from CEM simulations, as the effective Drude model of the gap medium almost resembles vacuum for large gap-widths. In contrast, for gap-widths <4 Å, the BDP resonance peak no longer red-shifts, and its intensity drops significantly. The BQP then becomes the dominant resonance in the spectra. Examination of Fig. 2a confirms that these features are indeed observed in the experiments for dimers with gap-widths <6.7 Å. Some differences are observed between the measured resonance peak positions and those predicted by QCM simulations. For example, the longest resonance wavelength predicted by the QCM simulations is ~1,050 nm, while the experimentally measured value is ~920 nm. This could be due to other quantum mechanical effects (such as nonlocality [9] , [11] ) that could occur at these very small gap-widths (see Supplementary Fig. 6 and Supplementary Note 2 for details). For dimers made of gold, it has been suggested that nonlocal effects would introduce a blue-shift in the plasmonic resonance compared with that obtained from CEM simulations [26] . A numerical model that considers both tunnelling and nonlocality would thus be preferred but is out of the scope of this report. Nevertheless, the QCM simulations explain the marked variation in the measured scattering spectra with gap-width, confirming electron tunnelling is the dominant quantum mechanical effect for the fabricated dimers with single-digit angstrom gap-width. Impact of electron tunnelling on plasmonic enhancement To investigate the impact of electron tunnelling on the near-field enhancement of dimers with atomic length-scale gaps, we perform SERS measurements, as SERS enhancement factor (EF) scales roughly as the fourth power of the near-field enhancement [27] . The results for two representative dimers (Dimer II and III in Fig. 1 ) are shown in Fig. 3 . From the far-field optical measurements and high-resolution TEM images, we conclude that electron tunnelling is expected for Dimer II, but not for Dimer III. For the SERS measurements, self-assembled monolayers (SAMs) of thiophenol are formed on the dimers. Thiophenol SAMs act as dielectric layers that overcoat all the exposed surfaces of dimers, that is, the top surfaces and the side walls, as revealed by TEM characterizations ( Supplementary Fig. 7 and Supplementary Note 3 ). We record the dark-field scattering spectra of the dimers with and without thiophenol SAMs. 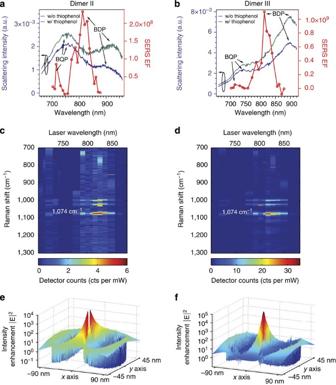Figure 3: Dark-field scattering and wavelength-scanned SERS measurements on Dimer II and III. (a,b) Dark-field scattering spectra measured before and after formation of thiophenol SAM, along with the measured wavelength-dependent SERS EFs, for Dimers II and III, whose gap-widths are 2.0 Å and 6.7 Å, respectively. Thiophenol Raman line of 1,074 cm−1is used to calculate SERS EFs. (c,d) Intensity maps of Raman scattering from Dimer II and III, respectively. Intensity is given by the detector counts normalized by laser power. (e) Near-field intensity distribution simulated by QCM for ideal nanodisc dimer structure with gap-width of 2.0 Å, at its BDP peak resonance wavelength. Intensity at the very centre of the gap is suppressed due to electron tunnelling. QCM predicts that maximum intensity is achieved at two hotspots just outside tunnelling gap region. (f) Near-field intensity distribution simulated by QCM for ideal nanodisc dimer structure with gap-width of 7 Å. Only one hotspot is observed at the centre of gap. Figure 3a,b shows that, for both dimers, SAM formation results in increased scattering intensities. The resonance lineshapes are maintained however. Of particular note is that the suppression of the BDP mode of Dimer II, compared with that of Dimer III, is maintained with the formation of the thiophenol SAM. This suggests that electron tunnelling through the SAM is still significant for such narrow gaps. Figure 3: Dark-field scattering and wavelength-scanned SERS measurements on Dimer II and III. ( a , b ) Dark-field scattering spectra measured before and after formation of thiophenol SAM, along with the measured wavelength-dependent SERS EFs, for Dimers II and III, whose gap-widths are 2.0 Å and 6.7 Å, respectively. Thiophenol Raman line of 1,074 cm −1 is used to calculate SERS EFs. ( c , d ) Intensity maps of Raman scattering from Dimer II and III, respectively. Intensity is given by the detector counts normalized by laser power. ( e ) Near-field intensity distribution simulated by QCM for ideal nanodisc dimer structure with gap-width of 2.0 Å, at its BDP peak resonance wavelength. Intensity at the very centre of the gap is suppressed due to electron tunnelling. QCM predicts that maximum intensity is achieved at two hotspots just outside tunnelling gap region. ( f ) Near-field intensity distribution simulated by QCM for ideal nanodisc dimer structure with gap-width of 7 Å. Only one hotspot is observed at the centre of gap. Full size image The dark-field measurements show that the BDP peak positions can shift over a fairly broad wavelength range as the gap-width varies from the nanometer-scale to the angstrom-scale. To ensure that the maximum SERS enhancement is measured for each dimer, we perform wavelength-scanned SERS measurements [28] (see Methods). The laser power is kept below 20 μW to avoid damage to the sample, thereby permitting multiple SERS measurements. It also avoids the nonlinear field enhancement that has been predicted to occur at higher intensities [29] , [30] . Each column of measurements in Fig. 3c,d shows the Raman intensity normalized by the laser power. The SERS EFs of the 1,074 cm −1 line for each laser wavelength is quantified for the two dimers, as shown in Fig. 3a,b . The results show that the wavelength-dependent SERS EF follows the lineshape of the dark-field scattering spectra but are blue-shifted, which is consistent with what has been reported previously [28] . The maximum SERS EF for Dimer II with 2.0 Å gap is 2.4 × 10 8 , achieved at the laser wavelength of ~815 nm. The maximum SERS EF for Dimer III with 6.7 Å gap is 1.2 × 10 9 , achieved at the laser wavelength of ~820 nm. These two measurements suggest that as gap-widths reduce to the single-digit angstrom range, the SERS EF, hence the field enhancement, does not increase as predicted by CEM [8] , but instead decreases. To further explain this observation, we simulate the electric field intensity distributions for dimers with gap-widths of 2 and 7 Å using the QCM ( Fig. 3e,f , respectively). For the dimer with a larger gap-width of 7 Å, Fig. 3f shows that only one hotspot occurs in the narrowest region of the gap, consistent with the near-field distribution of plasmonic dimers in the classical model [6] , with the maximum intensity enhancement being 7.0 × 10 4 . In contrast, Fig. 3e shows that QCM simulations predict a significant reduction in the near-field when the gap-width is 2 Å, with a smaller maximum intensity enhancement of 1.1 × 10 4 . The intensity distribution shows two hotspots, and the field at the centre of the gap is significantly suppressed. For dimers with such small gap-widths, the effective ‘charge-transfer' channel due to electron tunnelling becomes appreciable, thus reducing the build-up of charges of opposite signs on the two sides of the gap [12] , [30] . Further decrease in the gap-width after the emergence of electron tunnelling would thus reduce the field enhancement within the gap. Further evidence is shown in Fig. 4a , in which we analyse the results of the wavelength-scanned SERS measurements performed on 45 different dimers whose gap-widths range from 9.1 nm to 2.0 Å. For comparison, we use both CEM and QCM simulations to estimate the electromagnetic SERS EFs as shown in Fig. 4b . There are clearly two regions in Fig. 4a that show opposite trends for measured SERS EFs at 1,074 cm −1 Raman line as a function of gap-width. Similar trends are also observed for measured SERS EFs at 1,002 cm −1 Raman line, indicating that the chemical enhancement is not the dominant reason for these observed effects ( Supplementary Fig. 8 ). For gap-width ranging from 10 nm to 6.7 Å, it is observed that the SERS EF generally increases as the gap-width decreases, as expected by both CEM and QCM simulations shown in Fig. 4b . As gap-width decreases from 6.7 to 2.0 Å, the measured SERS EF no longer increases, but instead decreases significantly. Two models are used for CEM simulations: the CEM simulations of Model 1 assume monolayer coverage of the thiophenol molecules on the gold surfaces, as indicated by Supplementary Fig. 7 ; the CEM simulations of Model 2 consider the hypothetical case for which the thiophenol molecules cannot access the narrowest regions of the gap (see Supplementary Fig. 9 and Supplementary Note 3 for more details). Note that for gap-widths in the same range, both Model 1 and Model 2 CEM simulations still predict a monotonic increase of SERS EF as the gap narrows, which contradicts our observations. In contrast, the QCM simulations take into account electron tunnelling and predict a turning point around 4 Å in the SERS EF vs gap characteristics, in a similar manner to what is observed experimentally. Moreover, this range of gap-widths is in agreement with those for which we observe the impact of electron tunnelling on the dark-field scattering spectra of the same group of dimers. The emergence of electron tunnelling not only reduces the scattering intensity of the BDP mode, but also reduces the SERS EF. Through the correlation between the structures and the optical properties of dimers with angstrom-scale gaps, we thus demonstrate that the maximum achievable SERS EF, hence plasmonic field enhancement, is limited by the quantum mechanical electron tunnelling. 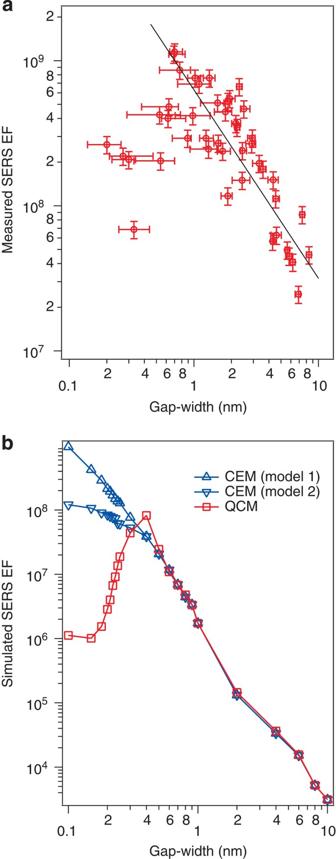Figure 4: Impact of quantum mechanical electron tunnelling on SERS EF. (a) Maximum SERS EFs for 45 dimers measured by wavelength-scanned SERS, shown as red circles. The horizontal error bars represent the errors in gap-width determination, which is retrieved following the procedures inSupplementary Note 1. The vertical error bars represent the errors in measuring SERS EFs, which is calculated from the uncertainties in reference Raman measurements for neat thiophenol (Supplementary Note 4). The gap-widths range from (2.0±0.6) Å to (9.1±0.4) nm. The maximum SERS EF measured is (1.2±0.2) × 109for Dimer III with gap-width of (6.7±1.1) Å. Two regions that show opposite trends for SERS EF as function of gap-width are observed. For gap-width ranging from 6.7 Å to 9.1 nm, the measured SERS EF generally follows the phenomenological linear fit (in a log-log scale) as log(EF)=8.8−1.3log(gap-width). The SERS EF generally increases as the gap-width decreases in this region. As gap-width further decreases from 6.7 to 2.0 Å, the SERS EF does not increase, but instead decreases significantly. (b) Simulated SERS EFs using both QCM and CEM for gap-widths ranging from 1 Å to 10 nm. Only electromagnetic SERS EF is considered (see Methods), and the simulated EFs are 1–2 orders smaller than the measured values mainly due to SERS chemical enhancement32,33. The CEM simulations of Model 1 assume monolayer coverage of the thiophenol molecules on the gold surfaces. The CEM simulations of Model 2 consider the hypothetical case for which the thiophenol molecules cannot access the narrowest regions of the gap. Figure 4: Impact of quantum mechanical electron tunnelling on SERS EF. ( a ) Maximum SERS EFs for 45 dimers measured by wavelength-scanned SERS, shown as red circles. The horizontal error bars represent the errors in gap-width determination, which is retrieved following the procedures in Supplementary Note 1 . The vertical error bars represent the errors in measuring SERS EFs, which is calculated from the uncertainties in reference Raman measurements for neat thiophenol ( Supplementary Note 4 ). The gap-widths range from (2.0±0.6) Å to (9.1±0.4) nm. The maximum SERS EF measured is (1.2±0.2) × 10 9 for Dimer III with gap-width of (6.7±1.1) Å. Two regions that show opposite trends for SERS EF as function of gap-width are observed. For gap-width ranging from 6.7 Å to 9.1 nm, the measured SERS EF generally follows the phenomenological linear fit (in a log-log scale) as log(EF)=8.8−1.3log(gap-width). The SERS EF generally increases as the gap-width decreases in this region. As gap-width further decreases from 6.7 to 2.0 Å, the SERS EF does not increase, but instead decreases significantly. ( b ) Simulated SERS EFs using both QCM and CEM for gap-widths ranging from 1 Å to 10 nm. Only electromagnetic SERS EF is considered (see Methods), and the simulated EFs are 1–2 orders smaller than the measured values mainly due to SERS chemical enhancement [32] , [33] . The CEM simulations of Model 1 assume monolayer coverage of the thiophenol molecules on the gold surfaces. The CEM simulations of Model 2 consider the hypothetical case for which the thiophenol molecules cannot access the narrowest regions of the gap. Full size image Achieving smaller gap-widths has been a long-pursued goal in the realization of SERS substrates. Our observations, however, indicate that reducing gap-width for SERS applications is not always beneficial. This phenomenon is also likely to be of crucial importance for other plasmonic applications, such as optical manipulation [4] , four-wave mixing [31] , high-harmonic generation [6] and optical rectification [7] . Compared with other methods for the formation of dimers with angstrom-scale gaps, we believe the experimental platform shown here offers unique advantages for these studies. First, the dimer structures are fixed on the substrate thereby enabling high resolution structural and optical characterization to be performed and correlated. Second, the metallic surface is free from contaminants such as ligands [10] or electron-beam-induced carbon deposition [16] . Finally, the reproducible fabrication method can be used with any substrate, with silicon nitride membranes being used here solely for the purpose of TEM characterization. This platform could also pave the way for understanding quantum plasmonics in metallic nanostructures that are more elaborate than dimers, such as heptamers and higher-order oligomers. We also note that, although electron tunnelling should be avoided to achieve large plasmonic enhancement, by actively controlling the effect, for example, by the Fowler-Nordheim effect [29] , future applications of quantum plasmonics could be enabled. In conclusion, we have developed a top-down nanofabrication method that achieves lithographically fabricated plasmonic dimers with gap-width down to single-digit angstrom range. By comparing the dimer structures and their scattering properties, we demonstrate the emergence of electron tunnelling at optical frequencies for metallic nanostructures with such small gap-widths. Through observation of SERS enhancements, we experimentally demonstrate that the maximum achievable plasmonic enhancement is limited by quantum mechanical electron tunnelling. This runs counter to the long-held assumption that smaller gaps in plasmonic antennas are always beneficial for enhanced light–matter interactions. Finally, we anticipate that the unique experimental platform provided by this work could further the understanding of quantum mechanical effects in plasmonic systems and enable future applications of quantum plasmonics. Sample fabrication Metallic dimers are fabricated on high-quality silicon nitride (SiN) membrane windows (NX5025X, Norcada), each with frame size of 5 × 5 mm 2 , window size of 250 × 250 μm 2 and SiN thickness of 30 nm. Both EBL exposures are performed using an Elionix F-125 EBL system. The first exposure starts with locating the SiN window using the scanning electron microscope (SEM) capability of the Elionix F-125. Then, an array of nanodiscs, with diameters of 90 nm, is patterned such that the centre of the array matches the centre of the SiN window. The periodicity of the array is chosen 4 × 4 μm 2 to minimize the coupling between adjacent dimers. The array has an overall extent of 300 × 300 μm 2 , that is, slightly larger than the extent of the SiN window. Two cross-shape alignment marks are also patterned in this exposure. After resist development, titanium (1 nm) and gold (20 nm) are evaporated, and lift-off is performed in acetone. The second exposure is performed, aligned to the first. This consists of another array of nanodiscs, again with diameters of 90 nm. The locations of the nanodiscs are designed such that the two arrays, if aligned perfectly, would form an array of dimers with gap size ranging from −40 nm (that is, overlapped) to +40 nm, gradually increasing by 0.05 nm for each successive dimer from the lower left to the upper right corners of the array. Typical translational alignment errors are below 10 nm, and rotational errors are below 1 mrad. Dark-field scattering spectroscopy All optical measurements reported in this paper are performed before TEM characterization to avoid the possibility of carbon contamination. Experimental setups are shown in Supplementary Fig. 10 . White light from a halogen lamp is loosely focused on the dimer array. The illumination is linearly polarized along the dimer long-axis and incident at an angle of 65° from the normal to the substrate. An objective lens (× 50, NA=0.55) and a tube lens ( f =200 mm) are placed above the sample and produce a dark-field image of the plasmonic dimer array at the entrance slit of the spectrometer (Acton SP2300). The entrance slit assembly is then replaced with a precision pinhole with a diameter of 200 μm to select the light scattered by the individual plasmonic dimer under study. A long-pass filter (passes λ >532 nm) placed in front of the pinhole is used to remove effect of second order diffraction by the grating in the spectrometer. The dark-field spectrum S generated by the spectrometer is then recorded from 550 to 1,050 nm with a liquid-nitrogen-cooled CCD camera (Princeton Instruments Spec-10). The integration time is 30 s. A reference spectrum R is measured from the light scattered by a white-light reflectance standard (WS-1-SL, Ocean Optics). The background spectrum B is measured from a region on the SiN window that does not contain any dimers. The spectrum from the dimer under study is then calculated as ( S - B )/ R . Wavelength-scanned Raman spectroscopy Before SERS measurements, SAMs of thiophenol are formed on the plasmonic dimers. We measure SERS spectra at 19 different laser wavelengths (every 10 nm from 705–885 nm) for each dimer. This is performed using a home-built wavelength-scanned confocal Raman microscope (epi-configuration). A Ti:sapphire laser (Mira 900, Coherent) that is tunable from 700–900 nm and operating in continuous-wave mode is used as the Raman excitation source. For each wavelength, the beam from the Ti:sapphire laser is spatially filtered with a precision pinhole with diameter of 75 μm. The light transmitted by the pinhole is collimated by a lens to a diameter of ~3 mm, which overfills the back-aperture of the objective lens (× 100, NA=0.9). A short-pass filter is used to remove light that might be otherwise collected into the spectrometer by Rayleigh scattering. A pellicle beamsplitter (8:92 splitting ratio, CM1-BP108, Thorlabs) then directs ~8% of the laser beam onto the objective, which creates a near diffraction-limited laser spot on the sample. This laser power is kept below 20 μW to avoid damage to the sample, thereby permitting multiple SERS measurements. It also avoids the nonlinear field enhancement that has been predicted to occur at higher intensities [29] , [30] . The long-axis of the dimer under study is placed along the polarization of the laser. A piezo-stage then moves the dimer into the centre of the beam to maximize the intensity of Stokes scattering. This Stokes scattering is then collected by the same objective lens and transmitted by the pellicle beamsplitter with an efficiency of ~92%. It then passes through a long-pass filter to remove the laser line and is focused on the spectrometer entrance slit. The Raman spectra are then measured by the spectrometer, which is equipped with a liquid-nitrogen-cooled CCD. Integration times of 60 s are used. Wavelength-scanned reference measurements are also made on a 500-μm thick fluid chamber containing neat thiophenol, as shown in Supplementary Fig. 11 . The power is in the mW range to achieve good signal-to-noise ratio. The SERS EF for an individual plasmonic dimer at each wavelength is then calculated based on the method described in Supplementary Note 4 . TEM characterization High-resolution TEM images of the dimers are taken with a JEOL 2100 TEM microscope. These images are obtained after optical characterization is complete. This is due to the fact that we observe a gradual accumulation of carbon on the dimers when the sample is within the TEM chamber. Before performing TEM imaging, the substrate is resized to be a circle with diameter of ~3 mm to fit into the TEM sample holder. This is done by gluing a molybdenum support ring with diameter of ~3 mm on the substrate and scribing away the unwanted part. TEM images are taken at an accelerating voltage of 200 kV and at magnifications of × 40,000 and × 400,000. A double-tilting TEM holder is used to avoid parallax. The sample is placed such that the dimer long-axis is roughly aligned with one of the rotational axes of the TEM holder. Classical electromagnetic model CEM simulations are performed using a commercial software package (Lumerical) that implements the 3D finite-difference time-domain (FDTD) method. A gold dimer with specific gap-width is placed on top of a thin layer of SiN with thickness of 30 nm and refractive index of n =2. The gold dimer simulated here is formed by two nanodiscs with diameters of 90 nm and thickness of 20 nm. Gold is described by a Drude model, with ε ∞ =1, ω p =1.94 × 10 15 Hz, and γ =2.14 × 10 13 Hz. The titanium adhesion layer is modelled by two nanodiscs with diameters of 94 nm ( Supplementary Fig. 5 ) and thicknesses of 1 nm. These are situated beneath the gold nanodiscs. The dielectric function of titanium is from a multi-coefficient fitting model provided by Lumerical FDTD. The symmetry in the plane of the substrate is exploited to minimize the simulation workload. A total-field scattered-field (TFSF) source simulates a linearly polarized plane wave normally incident on the dimer. Although this incidence angle is different from the dark-field scattering measurement, the difference in resonance intensity and peak wavelengths is minor ( Supplementary Fig. 12 ). Two power monitors that are placed outside the TFSF region measure the scattering spectrum of the dimer. A box that encloses the dimer structure has a uniform mesh of 0.5 nm. The mesh generated outside the box is non-uniform. For gaps narrower than 1 nm, a refined mesh area is generated within the gap region such that the gap width equals four unit cells. A 3D monitor having the same dimensions as the uniform mesh box records all field data within the box. These data are used for calculating the SERS EF shown in Fig. 4 . The surface-averaged SERS EF is given by , where the surface A includes all the surfaces that are 0.5 nm away from both the top surfaces and side walls of the dimer. Quantum-corrected model The Drude model that models the electron tunnelling and tunnelling conductivity within the gap is given by ref. 13 : where d is the gap distance. The effective plasma frequency ω g is chosen to be equal to that of gold. The effective damping frequency γ g is related to the tunnelling current and is given by where q =1.12 × 10 10 m −1 is the effective decay rate for gold dimers obtained from a phenomenological linear fit to the full quantum mechanical simulation data [13] . The gap region of the nanodisk dimer is then quantized into 8 effective layers of blocks with 8 different values of d . In addition to the mesh configurations for CEM simulations, a uniform mesh box with a grid cell size of 0.1 nm is added to enclose the region containing the Drude-like material that models the tunnelling. The configuration of field monitors is the same as that used in the CEM simulations. How to cite this article: Zhu, W. & Crozier, K. B. Quantum mechanical limit to plasmonic enhancement as observed by surface-enhanced Raman scattering. Nat. Commun. 5:5228 doi: 10.1038/ncomms6228 (2014).